Evidence for a difference in rupture initiation between small and large earthquakes The process of earthquake rupture nucleation and propagation has been investigated through laboratory experiments and theoretical modelling, but a limited number of observations exist at the scale of earthquake fault zones. Distinct models have been proposed, and whether the magnitude can be predicted while the rupture is ongoing represents an unsolved question. Here we show that the evolution of P-wave peak displacement with time is informative regarding the early stage of the rupture process and can be used as a proxy for the final size of the rupture. For the analysed earthquake set, we found a rapid initial increase of the peak displacement for small events and a slower growth for large earthquakes. Our results indicate that earthquakes occurring in a region with a large critical slip distance have a greater likelihood of growing into a large rupture than those originating in a region with a smaller slip-weakening distance. The slow, stable nucleation phase and its transition to a dynamic earthquake rupture have been thoroughly investigated by theoretical, numerical and laboratory studies to understand the preparatory phase of earthquakes and their potential to grow into a large event [1] , [2] , [3] , [4] , [5] , [6] . Being able to predict the final size of an earthquake while the rupture is ongoing on the fault plane is a highly debated scientific problem. Contrasting views have been proposed on whether the initial stage of the rupture process is different for small and large earthquakes [7] , [8] , [9] , [10] , [11] . According to the “cascade model”, the rupture starts in the same way for small and large earthquakes. The local friction conditions and the geometrical discontinuities of the fault surface control the final size [12] . The immediate implication of this model is that a seismic event is a stochastic process for which the final size cannot be known until the rupture has finished and is even more indeterminate when only the beginning of the process is considered. However, recent theoretical studies, seismic observations and laboratory experiments have indicated a possible scaling between the characteristics of the initiation phase and the earthquake magnitude, suggesting a potential deterministic nature of seismic rupture [13] , [14] , [15] , [16] . Ishihara et al . [7] analysed the moment rate function (MRF) of a few Japanese earthquakes and provided evidence for their different rising slopes, suggesting a causal relation between the MRF and the final event magnitude. Using a broader dataset, Ellsworth and Beroza [9] found that the size and duration of the initiation phase scale with the final magnitude. Several authors, in contrast, did not observe a change in the P-wave onset or they provided an alternative interpretation of the differences in the nucleation phase due to the filtering procedure or propagation effects [8] , [10] , [11] . The interest in rupture initiation was raised again recently because of its immediate impact on the rapid assessment of earthquake size. The ability to correctly distinguish a small shock from a large event through the analysis of the first P-wave observation is crucial for risk mitigation actions triggered by earthquake early warning systems. Several authors demonstrated that the early portion of recorded P-waves contains information regarding the magnitude through its frequency content and/or amplitude [17] , [18] , [19] , [20] . Most of these studies concentrated on the analysis of a fixed P-wave time window (PTW; 3–4 s). In the present study, we measure the peak displacement amplitude of filtered P-wave signals ( P d ) over a progressively expanding PTW. Previous studies of the beginning of waveforms analysed either a few earthquakes recorded at a limited number of stations or earthquakes belonging to the same sequence. Under such conditions, recognizing and clearly discriminating between source and propagation effects, both of which can influence the initial shape of signals, can be difficult. Here, we use a larger, high-quality dataset of 43 moderate-to-strong Japanese events spanning wide magnitude ( M ) and distance ( R ) ranges (4≤ M ≤9; 0≤ R ≤500 km). We analyse more than 7000 three-component waveforms recorded at 1,208 stations. 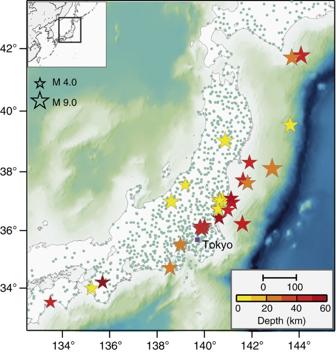Figure 1: Event map. The distribution of stations used in this study (small green circles) and the epicentral locations of the 43 selected events (coloured stars). The size of the star is proportional to the magnitude, and the colour represents the source depth. The black bar at the bottom right denotes a 100 km length. The full list of analysed events is provided in Supplementary Table 1 , while further details regarding the database selection are provided in the Supplementary Methods section. Figure 1 shows the map of stations used and the epicentres of the selected events. Figure 1: Event map. The distribution of stations used in this study (small green circles) and the epicentral locations of the 43 selected events (coloured stars). The size of the star is proportional to the magnitude, and the colour represents the source depth. The black bar at the bottom right denotes a 100 km length. Full size image Time evolution of peak displacement The number of analysed earthquakes ensures adequate data sampling in both magnitude and distance bins ( Fig. 2a–c ). For each event, the logarithm of P d versus PTW curve (hereafter abbreviated as LPW curve) is obtained by averaging the data from all available stations at any time (typically more than 100; see the Methods section). We found that each curve progressively increases with time until a final, stable value is reached. The plateau level (PL) and saturation time generally increase with magnitude ( Fig. 3a ). 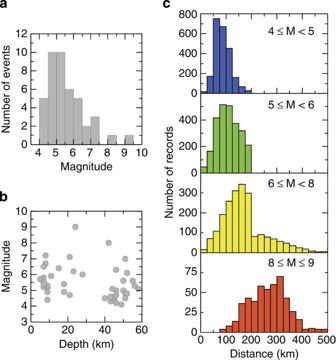Figure 2: Data histograms. (a) Histogram of the number of earthquakes as a function of magnitude. (b) Distribution of magnitude as a function of depth for the selected events. (c) Distribution of records as a function of distance for different magnitude classes. Figure 2: Data histograms. ( a ) Histogram of the number of earthquakes as a function of magnitude. ( b ) Distribution of magnitude as a function of depth for the selected events. ( c ) Distribution of records as a function of distance for different magnitude classes. 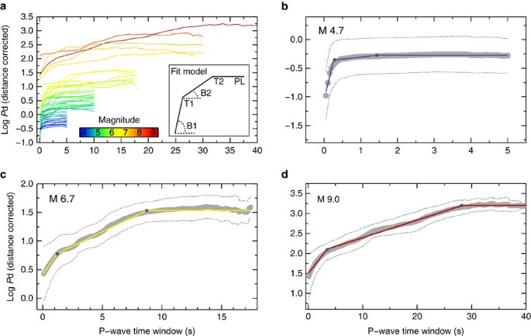Figure 3: LPW curves and model fit. (a) Average logarithm of thePdversus PTW (LPW) curve for each analysed event. They-axis represents the average logarithm ofPd, obtained by using all the available data at each time point, after correcting individual values for the distance effect (using equation 1). The insert box is a schematic representation of the piecewise linear fitting function. (b,c,d), Example of LPW curve for three representative events of magnitudeM4.7 (b), 6.7 (c) and 9 (d), respectively. In each panel, grey circles are the observed data with the associated ±1σ error bars (dashed lines). The solid line is the best fit function, obtained using the piecewise linear model and the dark squares mark T1 and T2 times of each event. Full size image Figure 3: LPW curves and model fit. ( a ) Average logarithm of the P d versus PTW (LPW) curve for each analysed event. The y -axis represents the average logarithm of P d , obtained by using all the available data at each time point, after correcting individual values for the distance effect (using equation 1). The insert box is a schematic representation of the piecewise linear fitting function. ( b , c , d ), Example of LPW curve for three representative events of magnitude M 4.7 ( b ), 6.7 ( c ) and 9 ( d ), respectively. In each panel, grey circles are the observed data with the associated ±1σ error bars (dashed lines). The solid line is the best fit function, obtained using the piecewise linear model and the dark squares mark T1 and T2 times of each event. Full size image For a single station, the far-field source kinematic models indicate that the P d versus time curve reproduces the shape of the apparent source time function [21] . By averaging P d among many stations, distributed over azimuth and distance, the resulting function approximates the MRF. Assuming a triangular shape for the MRF, the plateau of P d versus time curves is reached at the peak of the MRF, and the corresponding time is a proxy for the source moment and duration [22] . Our observations indicate that the initial shape of the P d versus time curves typically follows an exponential trend. Model fit for parameter estimation To reproduce the observed shape, we modelled the LPW curve using a piecewise linear function ( Fig. 3a , small box). For each event, we fit the data and determined the corner time of the first and second straight line (T1 and T2, respectively), the slope of the two lines (B1 and B2, respectively) and the final PL. Examples of fitted curves for three representative events are shown in Fig. 3b–d . As expected, T2 and PL scale with the magnitude ( Supplementary Fig. 1 ), which is an a posteriori validation of the hypothesis that averaged LPW curves approximate the MRF. Our main focus here is on T1 and B1 for their possible relation with the beginning of the rupture process. We found a significant log-linear correlation with magnitude for both T1 and B1. In particular, T1 increases with magnitude, whereas B1 is inversely proportional to the earthquake size ( Fig. 4a,b ). These results indicate that the evolution of the LPW curve at the early stage of the rupture is to some degree related to the final earthquake size. 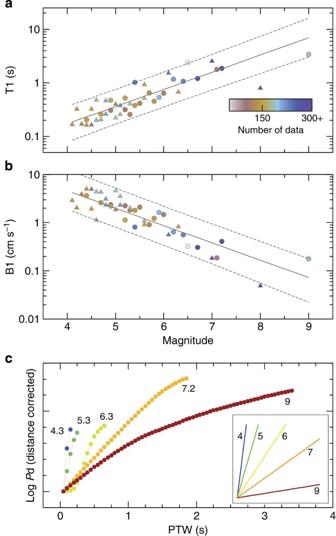Figure 4: Fit parameters T1 and B1. (a) First-corner time of the linear piecewise fit model as a function of magnitude for all the analysed events on a log-linear scale. The colour scale indicates the number of data points used for the average computation at time T1. (b) Slope of the first-line segment of the fit model as a function of magnitude for all the analysed events on a log-linear scale. For each individual B1 value, the colour is the same as that used inafor the corresponding T1 data point. Inaandb, small circles represent the crustal events (source depth <30 km), and triangles represent the subcrustal events (source depth⩾30 km). The solid grey line shows the linear best fit function, and the dashed lines are the 95% confidence intervals for new observations given the existing fit to the data. Error bars for individual data points are smaller than the symbol size. (c) Magnification of the LPW curve until time T1 for representative events. A common initial value has been assigned to compare the shape of the curves. The insert box shows the expected initial slope of the LPW curve for different magnitudes given the observed trend of B1 with magnitude. Figure 4c shows the observed LPW curve up to its T1 time for a few representative events and the expected slopes given the B1 versus magnitude trend (small box). The individual estimated parameters are remarkably accurate in terms of errors, and their scaling with magnitude is robust (linear correlation coefficient R 2 =0.8), although a clear variability appears in the plot of the whole dataset. Figure 4: Fit parameters T1 and B1. ( a ) First-corner time of the linear piecewise fit model as a function of magnitude for all the analysed events on a log-linear scale. The colour scale indicates the number of data points used for the average computation at time T1. ( b ) Slope of the first-line segment of the fit model as a function of magnitude for all the analysed events on a log-linear scale. For each individual B1 value, the colour is the same as that used in a for the corresponding T1 data point. In a and b , small circles represent the crustal events (source depth <30 km), and triangles represent the subcrustal events (source depth ⩾ 30 km). The solid grey line shows the linear best fit function, and the dashed lines are the 95% confidence intervals for new observations given the existing fit to the data. Error bars for individual data points are smaller than the symbol size. ( c ) Magnification of the LPW curve until time T1 for representative events. A common initial value has been assigned to compare the shape of the curves. The insert box shows the expected initial slope of the LPW curve for different magnitudes given the observed trend of B1 with magnitude. Full size image Tests and analyses of robustness Different factors might have influenced the shape of the LPW curves. The earthquake depth, for example, may impact source processes and frictional properties, thus affecting our observation regarding the evolution of P-wave peak displacement with time. Among the other factors, the high-pass filtering operation and the propagation effects related to crustal structure, geometrical spreading and anelastic attenuation are the most relevant. We performed different tests and separately investigated the influence of these factors on the analysis (see Supplementary Discussion and Supplementary Figs 2–6 for details). We did not find any clear evidence that either the source depth or the other effects are responsible for the observed trends of T1 and B1 with magnitude. Finally, we tested the persistence of the B1 trend with magnitude by limiting all the LPW curves to a fixed time window. We selected 1 s for M ⩾ 6 and 0.1 s for M <6, and for each event, we estimated the initial slope (by fitting data with a single straight line). Supplementary Fig. 7 shows that the slope estimates obtained within fixed time windows are consistent with those obtained by fitting the whole curves and that the trend of B1 with magnitude is still observed when only the very beginning of the curve is considered. Abrupt variations in the slip acceleration at the early stage of the rupture are associated with the unstable behaviour of the nucleation phase, before the onset of dynamic rupture propagation [23] . The characteristic time for the nucleation of large earthquakes is from one to a few seconds [15] , which is comparable to our estimates of the T1 time from the LPW curves ( Fig. 4a ). In the framework of linear slip-weakening models, analytical solutions of the nucleation phase indicate that the exponential growth is mainly controlled by the weakening rate [24] , [25] , which is the ratio between the strength drop of the fault related to the friction and the characteristic slip-weakening distance (D c ) over which the energy is dissipated. During nucleation, the initial stress is close to the threshold in the slipping zone. We can therefore replace the strength drop with dynamic stress drop in our interpretation. Observations indicate a decrease in B1 of approximately one order of magnitude in the range M 4.5–7 ( Fig. 4b ). In the same range, this decrease would correspond either to a decrease in the initial stress or to an increase in the critical slip distance, both of one order of magnitude. Far-field measurements indicate an unclear scaling, or eventually a weak increase, in the stress drop with magnitude in this range [26] . Although these estimates refer to the whole rupture process, an initial decrease is unlikely to result in a final constant value, independent of magnitude. In contrast, assuming for D c a characteristic value of 0.5–1 m for an M =7 event [27] , the corresponding value for an M =4.5 event would be at the scale of 5–10 cm. Extrapolating this value to negative magnitudes, micrometric-to-millimetric values for D c would be obtained, consistent with the estimates from laboratory experiments. Such a scaling indicates the availability of a larger fracture energy in the initial stage of the rupture for larger magnitude events. In addition, the nucleation size is directly linked to the weakening rate for linear slip-weakening models [28] , which suggests a larger size and a longer characteristic time of the nucleation of larger events, as confirmed by the positive scaling of T1 with magnitude. Increasing in the breakdown energy with magnitude is commonly interpreted in earthquake fracture mechanics as a homogenized effect of all competing dissipative mechanisms on the fault plane, such as friction, off-fault damage, thermal pressurization and melting [29] . Extending this interpretation to the initial stage of the rupture, possible changes in D c along the fault can be related to a characteristic length of the asperities [3] or to an intrinsic stiffness of the fault zone, which elastically accumulates energy during tectonic fault loading. Assuming a variable, fractal distribution of the D c on the fault, with some space coherency, we argue that when an earthquake rupture develops over a region with a low D c value, its probability of rupturing adjacent regions is low. In contrast, when a coherent rupture nucleates in a region of larger D c , the probability that it will grow into a larger size event increases. In this context, the variation of D c and of the probability that an initial earthquake rupture will grow justifies the dispersion of B1 values with respect to magnitude. Finally, the log-linear relationship between the MRF and B1 indicates the exponential growth of the nucleation phase. Although the observed T1 values are comparable to the nucleation times, we cannot exclude the possibility that they involve the initial acceleration of the dynamic rupture phase. In addition, larger breakdown energy prevents a rapid acceleration of the rupture at this initial stage, which also limits the moment rate increase with time. The observed variation in B1 with magnitude may have an important impact on the rapid assessment of the earthquake size. Nevertheless, the slope measured in this work is derived from the average trend of hundreds of records, spanning wide azimuth and distance ranges, whereas in real-time, the availability of data depends on the source-station geometry. Further analyses are therefore required to simulate the real-time data streaming and to assess the minimum near-source data necessary to constrain the initial slope. Assuming that the slope is well-constrained from near-source data, a short time window (approximately 1 s, Supplementary Fig. 7 ) is sufficient for an evaluation of the earthquake size. Data processing and average peak displacement computation To obtain displacement waveforms, the mean value and linear trend are first removed from the raw acceleration data. These records are then double integrated, and a non-causal, high-pass Butterworth filter with a cutoff frequency of 0.075 Hz is applied to remove the artificial long-period trend and baselines introduced by the double-integration operation. The P-wave onset times were manually selected from each vertical component of the accelerometer records. We measured the peak displacement amplitude on the filtered P-wave signals ( P d ) over a progressively expanding PTW, starting from 0.05 s after the P-wave onset time and continuing until the expected arrival of the S-phase [30] . For each event, we obtained the LPW curve by averaging all the available data at each time window after correcting the observed P d values at different stations for the geometrical attenuation effect. To compare the observed P d values at different stations, the geometrical attenuation effect was corrected with the following attenuation relationship: where M is the event magnitude, P d is measured in cm (in a fixed time window of 3 s) and the hypocentral distance R is measured in km. In equation (1), a single term (log R ) is used to account for both the geometrical spreading and the anelastic attenuation. The magnitudes used here are provided by Japan Meteorological Agency and are assumed to be equivalent to moment magnitudes. For earthquakes with M <7, we used only data up to a maximum hypocentral distance of 200 km, whereas for M ⩾ 7 events, we included records up to 500 km. We preliminarily estimated the coefficients A , B and C of equation (1) for each distance range through a non-weighted linear regression analysis. Then, depending on the magnitude and the distance range, we used the appropriate coefficients to compare the observed P d values at different stations. Supplementary Table 2 shows the coefficients A , B and C for each magnitude and distance range. To avoid the inclusion of S-waves in the considered PTW, we computed the expected S-wave arrival time at each station ( T s ) using the following relation: where T p is the observed P-wave onset time, R is the hypocentral distance in km and b =0.088. The coefficient b was derived through a linear regression analysis after manually selecting the S-wave arrival times for a limited number of records from our dataset. For each event, we set a maximum PTW to be explored, based on the expected duration of the source from kinematic models for the corresponding magnitude, and considered at least twice the expected duration. To compute the average LPW curve, we also required at least five data points to be used in each PTW. The average computation stops either when the number of data points is not sufficient or when the PTW reaches its maximum time limit, whichever condition occurs first. To model the LPW curves, we used a piecewise, linear fit function inverted for five unknown parameters: first- and second-corner times (T1 and T2, respectively), the slope of the two straight lines (B1 and B2, respectively) and the final PL. How to cite this article: Colombelli, S. et al . Evidence for a difference in rupture initiation between small and large earthquakes. Nat. Commun. 5:3958 doi: 10.1038/ncomms4958 (2014).